Evolution of separate predation- and defence-evoked venoms in carnivorous cone snails Venomous animals are thought to inject the same combination of toxins for both predation and defence, presumably exploiting conserved target pharmacology across prey and predators. Remarkably, cone snails can rapidly switch between distinct venoms in response to predatory or defensive stimuli. Here, we show that the defence-evoked venom of Conus geographus contains high levels of paralytic toxins that potently block neuromuscular receptors, consistent with its lethal effects on humans. In contrast, C. geographus predation-evoked venom contains prey-specific toxins mostly inactive at human targets. Predation- and defence-evoked venoms originate from the distal and proximal regions of the venom duct, respectively, explaining how different stimuli can generate two distinct venoms. A specialized defensive envenomation strategy is widely evolved across worm, mollusk and fish-hunting cone snails. We propose that defensive toxins, originally evolved in ancestral worm-hunting cone snails to protect against cephalopod and fish predation, have been repurposed in predatory venoms to facilitate diversification to fish and mollusk diets. Venomous marine gastropods of the genus Conus have evolved one of the most sophisticated envenomation strategies known, allowing these slow animals to capture worms, mollusks and even fish [1] . Utilizing a hollow, harpoon-like radula, cone snails inject a complex cocktail of potent venom peptides (conotoxins) to rapidly immobilize the prey [2] . This strategy is underpinned by a remarkable diversity of conotoxins that target a wide range of membrane proteins, including the FDA-approved Ca v 2.2 inhibitor ω-MVIIA (Prialt) used to treat intractable pain [3] . To maximize venom potency, cone snails deploy synergistic groups of conotoxins, known as ‘cabals’ [4] . For example, the ‘lightning-strike cabal’ comprises potassium channel blocking κ-conotoxins and excitatory sodium channel modifying δ-conotoxins that produce immediate tetanic paralysis in fish [2] . In contrast, the ‘motor cabal’ developed in particular by C. geographus comprises inhibitory ω-, μ- and α-conotoxins that target neuromuscular receptors and produce flaccid paralysis in fish [5] . However, the role of the paralytic motor cabal in C. geographus predation is unclear, since it mainly uses an alternate ‘nirvana cabal’ to sedate fish prior to capture using a net strategy (see Supplementary Fig. 1 ; Supplementary Movie 1 ) [6] . Molecular and phylogenetic studies have demonstrated that the evolution of envenomation strategies is typically a predatory rather than a defensive adaptation [7] , [8] , despite the critical importance of defence for animal survival [9] . While a shell can serve as the first line of defence, repair marks commonly observed in many Conus species indicate they can survive physically damaging attacks from predators such as octopus or fish (see Supplementary Fig. 2 ), possibly by using their venom defensively (see Supplementary Movie 2 ). The defensive use of venom can also result in human injuries, with Conus geographus stings producing confirmed fatalities [5] . Such deleterious effects are currently explained by a unique venom that acts on targets with conserved pharmacology across prey and predator, and a separately evolved defensive strategy to deter aggressors has not been investigated previously. In this article, we report for the first time the remarkable ability of cone snails to rapidly and reversibly switch between functionally and structurally distinct venoms in response to predatory or threatening stimuli. The defence-evoked venom typically comprises paralytic toxins, previously thought to participate in prey capture, that explain the symptoms associated with human envenomation. In contrast, the predation-evoked venom appears largely devoid of these paralytic toxins. The venom duct shows a corresponding regionalization of toxin production, with high levels of defence-evoked and predation-evoked venoms in the proximal and distal sections, respectively. Finally, molecular evolution analyses revealed that both predatory and defensive toxins are evolving under strong positive selection. Together, these data suggest that ancestral defensive toxins originally evolved to protect against fish and cephalopod predators facilitated a shift from worm-hunting to fish- and mollusk-hunting strategies. Distinct predation- and defence-evoked venoms in cone snails Fish-hunting C. geographus possesses one of the most fragile shells ( Supplementary Fig. 3 ) and produces arguably the most potent venom, suggesting that reduced protection may have co-evolved with a highly developed defensive strategy in cone snails. To investigate the evolution of predatory and defensive envenomation strategies in cone snails, we developed a new method that allowed the sequential collection of injected venom from individual C. geographus using alternating predatory and defensive stimuli ( Supplementary Fig. 4 ). Surprisingly, the defence-evoked venom was significantly more complex than predation-evoked venom ( Fig. 1a–c ), with limited overlap in peptide composition (<50%), indicating that defence- and predation-evoked venoms are produced by distinct and independently controlled mechanisms ( Fig. 1d , Supplementary Fig. 5 ). The predation-evoked venom, which was injected only when the proboscis came in close proximity to appropriate prey tissue, lacked most of the paralytic peptides thought to enable prey capture but instead contained high levels of the fish-specific sodium channel inhibitor μ-conotoxin GS and non-paralytic peptides, including the vasopressin receptor agonist conopressin-G and the NMDA receptor antagonist conantokin G ( Supplementary Fig. 6 ). In contrast, paralytic peptides dominated the defence-evoked venom, which was injected immediately when the proboscis contacted a solid surface ( Supplementary Movie 3 ). 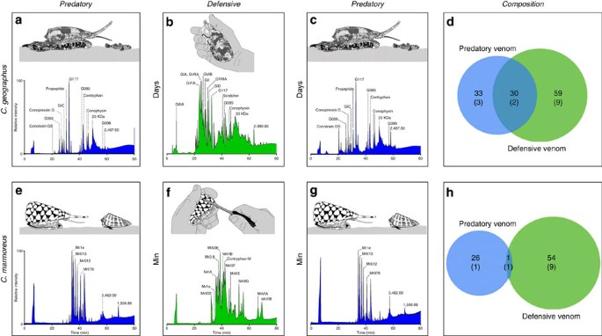Figure 1: The predation- and defence-evoked venoms of cone snails. (a–c) LC-MS profiles of venom samples collected from the deadly piscivorousConus geographusfollowing alternating predatory (a,c) and defensive (b) stimuli (milkings separated by 1–7 days). The two predation-evoked venom samples (clear venom), although interrupted by a defensive milking (milky venom with granules), were identical in composition and contained mainly the non-paralytic contryphan-G, conopressin-G, conophysin-G and a new conotoxin (G117). In contrast, the defence-evoked venom was more complex and contained paralytic conotoxins, including the presynaptic calcium channel blockers ω-GVIA, ω-GVIB, ω-GVIIA, the postsynaptic muscle nicotinic receptor antagonists α-GI, α-GIA and α-GII, and the sodium channel inhibitor μ-GIIIA, which evidently are used to defend against predators rather than for prey capture, as previously believed. (d) Overall, <50% of the major predatory toxins are also injected in defence, mostly at significantly lower levels (the number of previously characterized toxins compared with the total number of major masses detected are shown in parenthesis). (e–g) Show similar data for the molluscivorousC. marmoreus, which can repeatedly inject venom over much shorter intervals than piscivorous species (minutes versus days). (h) Remarkably, the predation- and defence-evoked venoms ofC. marmoreusare even more divergent compared with the venom ofC. geographus. Again, the defence-evoked venom contained vertebrate-active neurotoxins, including χ-MrIA, μO-MrVIA and μO-MrVIB. Examining the number of previously characterized toxins revealed a bias towards the discovery of defensive toxins in previous studies (d,h). Figure 1: The predation- and defence-evoked venoms of cone snails. ( a – c ) LC-MS profiles of venom samples collected from the deadly piscivorous Conus geographus following alternating predatory ( a , c ) and defensive ( b ) stimuli (milkings separated by 1–7 days). The two predation-evoked venom samples (clear venom), although interrupted by a defensive milking (milky venom with granules), were identical in composition and contained mainly the non-paralytic contryphan-G, conopressin-G, conophysin-G and a new conotoxin (G117). In contrast, the defence-evoked venom was more complex and contained paralytic conotoxins, including the presynaptic calcium channel blockers ω-GVIA, ω-GVIB, ω-GVIIA, the postsynaptic muscle nicotinic receptor antagonists α-GI, α-GIA and α-GII, and the sodium channel inhibitor μ-GIIIA, which evidently are used to defend against predators rather than for prey capture, as previously believed. ( d ) Overall, <50% of the major predatory toxins are also injected in defence, mostly at significantly lower levels (the number of previously characterized toxins compared with the total number of major masses detected are shown in parenthesis). ( e – g ) Show similar data for the molluscivorous C. marmoreus , which can repeatedly inject venom over much shorter intervals than piscivorous species (minutes versus days). ( h ) Remarkably, the predation- and defence-evoked venoms of C. marmoreus are even more divergent compared with the venom of C. geographus . Again, the defence-evoked venom contained vertebrate-active neurotoxins, including χ-MrIA, μO-MrVIA and μO-MrVIB. Examining the number of previously characterized toxins revealed a bias towards the discovery of defensive toxins in previous studies ( d , h ). Full size image Similar predation- and defence-evoked venom profiles were obtained for several C. geographus specimens ( Supplementary Figs 5–7 ). To examine how broadly a separate defensive strategy has evolved in Conus species, we extended these studies to molluscivorous and vermivorous cone snail species. The molluscivorous Conus marmoreus can inject its prey multiple times during a single feeding event, allowing predation- and defence-evoked venoms to be collected over short time-intervals ( Fig. 1e–g ). The predatory- and defence-evoked venoms of C. marmoreus were again distinct, with the first and third injections (both predatory) being identical ( Fig. 1e,g ), despite an intervening defensive sting being collected minutes earlier ( Fig. 1f ). The occurrence of only trace amounts of major predatory toxins (for example, Mr1e) detected in the defence-evoked venom confirmed that there was minimal venom carryover between stings ( Fig. 1h ). As observed for C. geographus , the predation-evoked venom of C. marmoreus was relatively simple compared with its defence-evoked venom, which contained several known vertebrate-active neurotoxins ( Fig. 1e ). Since C. marmoreus is not known to prey on vertebrates, these results suggest that these vertebrate-active toxins have specifically evolved for defence. In contrast, neurotoxins previously thought to participate in prey capture are absent from the predation-evoked venom, including the μO-conotoxins that inhibit mollusk [10] and vertebrate sodium channels [11] . Confirming this is a widely evolved strategy on cone snails, complex defence-evoked venoms were also obtained from other fish- ( Conus obscurus ), mollusk- ( Conus victoriae ) and worm-hunting species ( Conus planorbis and Conus coronatus ) ( Supplementary Figs 8–10 ). Pharmacological profiles of predation- and defence-evoked venoms To further investigate the biological significance of separate envenomation strategies, we compared the biological activity of predation- and defence-evoked C. geographus venoms across human sodium and calcium channels, and nicotinic acetylcholine receptors. Our results confirmed that the defence-evoked venom contained high levels of paralytic peptides acting at mammalian ion channels ( Fig. 2a–h ), which likely account for the human fatalities associated with C. geographus defensive stings (up to ~6 mg venom injected per strike). In contrast, the predation-evoked venom of C. geographus was inactive at these human targets, except for calcium channel activity associated with trace amounts of the highly potent calcium channel blockers ω-GVIA and ω-GVIIA. Since C. geographus is a piscivorous species, a fish bioassay was used to determine the effective dose (ED 50 ) in vivo of both the predation- and defence-evoked venoms ( Supplementary Fig. 11 ). Defence-evoked venom was 350-fold more potent (ED 50 =10 μg kg −1 ) than the predation-evoked venom at producing paralysis in fish, consistent with its role in deterring large predators, although sufficient predation-evoked venom (~1 mg) was injected to rapidly paralyse fish up to 200 g. Surprisingly, one of the major and novel components of the predation-evoked venom (G117, Fig. 1a ) did not induce paralysis when injected in fish, although a role for this peptide in the ‘nirvana cabal’ cannot be excluded. 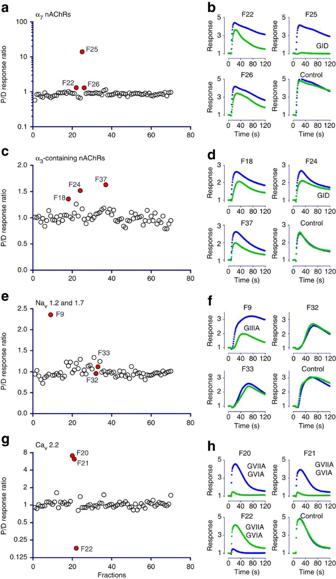Figure 2: Action of predation- and defence-evokedC. geographusvenoms on human receptors. (a–d) Both predation- (blue) and defence-evoked (green) venoms (1 mg each) were separated on RP-HPLC. The resulting 72 1-min fractions (F1-F72) were screened on SH-SY5Y human neuroblastoma cells for activity at α7 (a,b) and α3-containing nicotinic receptors (c,d), Nav1.2 and Nav1.7 voltage-gated sodium channel (e,f) and Cav2.2 voltage-gated calcium channel (g,h). Active fractions are highlighted in red on the left panels, with a response ratio >1 indicating greater activity in the defence than the predation-evoked venom, and vice versa (except F32 and F33, which show minor slowing of the response for Nav1.2/7 in both predation- and defence-evoked venoms). Specific responses for active fractions are shown on the right panels (b,d,fandh), and known toxins detected in these fractions are indicated. Whereas the predation-evoked venom only shows full inhibition of Cav2.2 response due to trace amount of ω-GVIIA and ω-GVIA, the defence-evoked venom shows potent inhibition of all molecular targets, with several well-characterized toxins identified in the active fractions. The potent block of these key physiological ion channels explains the lethal effect ofC. geographusdefensive envenomation on humans. Figure 2: Action of predation- and defence-evoked C. geographus venoms on human receptors. ( a – d ) Both predation- (blue) and defence-evoked (green) venoms (1 mg each) were separated on RP-HPLC. The resulting 72 1-min fractions (F1-F72) were screened on SH-SY5Y human neuroblastoma cells for activity at α7 ( a , b ) and α3-containing nicotinic receptors ( c , d ), Na v 1.2 and Na v 1.7 voltage-gated sodium channel ( e , f ) and Ca v 2.2 voltage-gated calcium channel ( g , h ). Active fractions are highlighted in red on the left panels, with a response ratio >1 indicating greater activity in the defence than the predation-evoked venom, and vice versa (except F32 and F33, which show minor slowing of the response for Nav1.2/7 in both predation- and defence-evoked venoms). Specific responses for active fractions are shown on the right panels ( b , d , f and h ), and known toxins detected in these fractions are indicated. Whereas the predation-evoked venom only shows full inhibition of Ca v 2.2 response due to trace amount of ω-GVIIA and ω-GVIA, the defence-evoked venom shows potent inhibition of all molecular targets, with several well-characterized toxins identified in the active fractions. The potent block of these key physiological ion channels explains the lethal effect of C. geographus defensive envenomation on humans. Full size image Origin of predation- and defence-evoked venoms The long, convoluted venom duct is the dominant toxin secretory organ in cone snails, but it is unclear if other embryologically related organs might also participate in venom production [12] . Analyses of the transcriptomes and proteomes of the interconnected venom gland, salivary gland and radular sac of C. geographus unequivocally demonstrated that both predation- and defence-evoked venoms arise from the venom duct and not these other associated tissues ( Supplementary Figs 12 and 13 ), with 127 conotoxin sequences recovered from the venom duct, including 43 confirmed by tandem mass spectrometry (MS/MS) ( Supplementary Table 1 ). In contrast, no conotoxin sequences were found in the salivary gland, and only three rare conotoxin transcripts were identified in the radula sac transcriptome, although these were not detected in the injected venoms. To understand how a single gland can rapidly and reversibly produce two distinct venoms, we analysed the venom peptide composition along the venom duct of C. geographus ( Fig. 3a–c ). Unexpectedly, the paralytic toxins found in the defence-evoked venom were abundant in the proximal duct (sections 7–12), whereas the major toxins found in the predation-evoked venom dominated the distal sections (sections 1–6 close to the pharynx) ( Fig. 3d , Supplementary Fig. 14 ). In addition, structural differences within the venom duct support the distinct partition of the gland producing toxins ( Fig. 3e ). These results suggest that stimulus-dependent spatiotemporal release of toxins from different segments of the venom duct can generate functionally and biochemically distinct predation- and defence-evoked venoms ( Fig. 3f ). 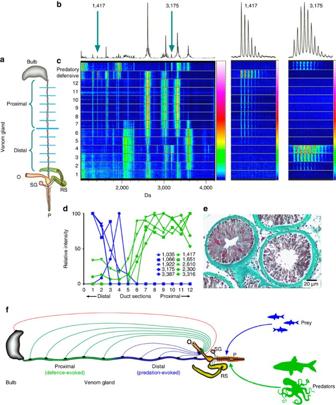Figure 3: Distribution of toxins inC. geographusvenom duct and proposed mechanism for venom release. (a) Twelve venom gland sections were spotted on a MALDI plate together with predation- and defence-evoked venom (O, oesophagus; P, proboscis; RS, radular sac; SG, salivary gland). (b) The resulting averaged spectrum is highly complex in the range 1,000–4,000 kDa corresponding to the size of most conotoxins (10–30 amino acids). (c) Gel view representation of MALDI results reveals distinct regionalization of many venom components along the duct. For example, the predatory toxin at 3,175 kDa and defensive toxin at 1,417 kDa show clear non-overlapping distribution along the duct. (d) Quantification of five major predatory (including conopressin-G at 1,035 kDa) and defensive (including α-GII at 1,417 kDa, μ-GIIIA at 2,610 kDa and ω-GVIIA at 3,316 kDa) toxins confirms this region-specific toxin production. (e) Histology (formaldehyde-fixed animal embedded in paraffin) reveals structural heterogeneity along the venom duct, including regions with a dense layer of secretory cells and a small lumen and others with a looser cell arrangement and a larger lumen, which could support such regional specialization. Gomori’s Trichrome stain shows muscle fibres in red, collagen in green and nuclei in blue/black (scale bar, 20 μm). (f) A simple hypothesis to explain the generation of separate stimulus-evoked venoms is proposed. An initial stimulus (predatory or defensive) is perceived by mechanical, visual and/or chemical (olfactory) sensors that transmit information to the cerebral ganglia surrounding the oesophagus (O) to activate two separate neuronal circuits. Predation-evoked stimuli activate neuronal circuit (blue) innervating the distal venom duct, causing the release of predatory venom peptides into the venom duct lumen. Similarly, threats including larger fish and cephalopods activate a separate defensive neuronal circuit (green) that innervates the proximal venom duct, causing the release of defensive toxins into the lumen. These lumen contents are then moved to the proboscis by a synchronized contraction of the muscular venom bulb to generate the injected ‘predation-evoked’ and ‘defence-evoked’ venoms. This key role of the venom bulb allows the rapid switch between the predation- and defence-evoked venoms observed. This mechanism of stimulus-dependent release of toxins from different sections of the venom duct explains how distinct predation- and defence-evoked venoms are generated. Figure 3: Distribution of toxins in C. geographus venom duct and proposed mechanism for venom release. ( a ) Twelve venom gland sections were spotted on a MALDI plate together with predation- and defence-evoked venom (O, oesophagus; P, proboscis; RS, radular sac; SG, salivary gland). ( b ) The resulting averaged spectrum is highly complex in the range 1,000–4,000 kDa corresponding to the size of most conotoxins (10–30 amino acids). ( c ) Gel view representation of MALDI results reveals distinct regionalization of many venom components along the duct. For example, the predatory toxin at 3,175 kDa and defensive toxin at 1,417 kDa show clear non-overlapping distribution along the duct. ( d ) Quantification of five major predatory (including conopressin-G at 1,035 kDa) and defensive (including α-GII at 1,417 kDa, μ-GIIIA at 2,610 kDa and ω-GVIIA at 3,316 kDa) toxins confirms this region-specific toxin production. ( e ) Histology (formaldehyde-fixed animal embedded in paraffin) reveals structural heterogeneity along the venom duct, including regions with a dense layer of secretory cells and a small lumen and others with a looser cell arrangement and a larger lumen, which could support such regional specialization. Gomori’s Trichrome stain shows muscle fibres in red, collagen in green and nuclei in blue/black (scale bar, 20 μm). ( f ) A simple hypothesis to explain the generation of separate stimulus-evoked venoms is proposed. An initial stimulus (predatory or defensive) is perceived by mechanical, visual and/or chemical (olfactory) sensors that transmit information to the cerebral ganglia surrounding the oesophagus (O) to activate two separate neuronal circuits. Predation-evoked stimuli activate neuronal circuit (blue) innervating the distal venom duct, causing the release of predatory venom peptides into the venom duct lumen. Similarly, threats including larger fish and cephalopods activate a separate defensive neuronal circuit (green) that innervates the proximal venom duct, causing the release of defensive toxins into the lumen. These lumen contents are then moved to the proboscis by a synchronized contraction of the muscular venom bulb to generate the injected ‘predation-evoked’ and ‘defence-evoked’ venoms. This key role of the venom bulb allows the rapid switch between the predation- and defence-evoked venoms observed. This mechanism of stimulus-dependent release of toxins from different sections of the venom duct explains how distinct predation- and defence-evoked venoms are generated. Full size image Defence as a major evolutionary force driving cone snail venom evolution To assess the influence of natural selection on conotoxins, we determined the non-synonymous to synonymous nucleotide substitution rate ratio (ω) and identified sites evolving under episodic bursts of positive Darwinian selection ( Supplementary Tables 2 and 3 ). Indeed, since the distinct distribution of toxins along a single venom gland is a unique evolutionary innovation, it could facilitate the separate evolution of specialized predatory and defensive venoms, which likely contributed to the rapid speciation observed in the genus Conus over the last 33 million years [13] . Our analyses detected a large number of positively selected sites (ω>1) in all toxin superfamilies examined, indicating that both predatory and defensive conotoxins are rapidly evolving under the influence of positive Darwinian selection ( Fig. 4a ). We also detected several lineages in the phylogenies of Conus defensive and predatory toxins that were influenced by episodic positive selection ( Supplementary Tables 2 and 3 ). Assessment of the widely distributed ancestral plesiotypic (ancestral character state) conotoxin superfamily O1 (ref. 14 ) highlights the distinct evolutionary trajectories adopted by C. geographus defensive and predatory toxins ( Fig. 4b ), with most of the characterized defensive toxins being found in a distinct clade separate from the predatory toxins. 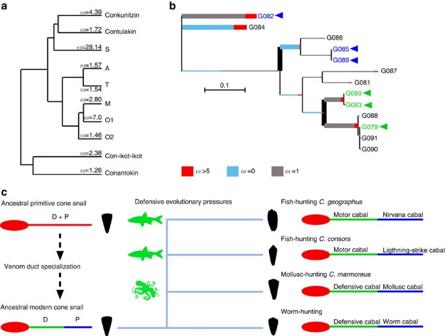Figure 4: Molecular evolution of conotoxin gene superfamilies and the role of defensive evolutionary pressure on cone snail venom evolution. (a) Molecular evolution assessment indicates that allC. geographusconotoxin superfamilies are rapidly evolving (ω>1). (b) Branch-site Random Effects Likelihood of superfamily O1 indicates the episodic nature of conotoxin evolution, revealing independent trajectories for defensive (green) or predatory (blue) conotoxins. (c) Specialization of the venom duct is a key evolutionary innovation in cone snails (venom duct and the associated proximal venom bulb are illustrated). We propose that the distinct defence (D) and predation-evoked (P) venoms found in the specialized venom ducts of modern cone snails evolved from an ancestral primitive cone snail that used the same venom produced in an unspecialized duct to deter predators and catch prey. This defensive behaviour, initially evolved to deter threats including cephalopod (octopus) and fish, likely triggered shifts in cone snail predatory strategies to mollusk- and fish-hunting that allowed predators to become prey. Figure 4: Molecular evolution of conotoxin gene superfamilies and the role of defensive evolutionary pressure on cone snail venom evolution. ( a ) Molecular evolution assessment indicates that all C. geographus conotoxin superfamilies are rapidly evolving (ω>1). ( b ) Branch-site Random Effects Likelihood of superfamily O1 indicates the episodic nature of conotoxin evolution, revealing independent trajectories for defensive (green) or predatory (blue) conotoxins. ( c ) Specialization of the venom duct is a key evolutionary innovation in cone snails (venom duct and the associated proximal venom bulb are illustrated). We propose that the distinct defence (D) and predation-evoked (P) venoms found in the specialized venom ducts of modern cone snails evolved from an ancestral primitive cone snail that used the same venom produced in an unspecialized duct to deter predators and catch prey. This defensive behaviour, initially evolved to deter threats including cephalopod (octopus) and fish, likely triggered shifts in cone snail predatory strategies to mollusk- and fish-hunting that allowed predators to become prey. Full size image In this study, we have discovered that the carnivorous gastropods of the genus Conus were able to rapidly and reversibly alternate between two distinct venoms in response to predatory or defensive stimuli. Surprisingly, defence-evoked venoms obtained from the deadly C. geographus contained high levels of paralytic conotoxins of the motor cabal, suggesting this cabal has evolved for defence and not for prey capture as previously suggested [5] . Consistent with a prominent defensive role for the motor cabal, the pharmacology of the defence-evoked venom correlates with the symptomatology following C. geographus envenomation in humans, with death typically resulting from respiratory paralysis [15] . In contrast, the predation-evoked venom contains prey-specific toxins that show low activity on human ion channels, indicating predation- and defence-evoked venoms have separately evolved for different functions. Expanding our study on the feeding mode of molluscivorous cone snails that routinely inject prey multiple times to achieve full paralysis, we have investigated the most behaviourally relevant milking sequence, where predatory use of venom is occasionally interrupted by deployment of defensive venom. The intervening defensive sting does not alter the composition and quantity of venom injected next, as the two separate predatory stings were strictly identical both qualitatively and quantitatively, with no evidence of depletion. Complex defence-evoked venom could also be obtained from other fish-hunting species, as well as from mollusk- and worm-hunting species, demonstrating that a specialized defensive behaviour and associated defensive venom has evolved widely across the genus Conus . Our transcriptomic and proteomic investigation of embryologically related organs revealed that the venom duct produced all conotoxins found in both predation- and defence-evoked venoms, with only three rare conotoxin transcripts retrieved from the radular sac, and no conotoxin-like sequences found in the salivary gland. However, while these rare transcripts likely have no current functional role, we cannot exclude an ancestral role in conotoxin evolution given they have the canonical organization of conotoxin precursors (signal peptide, propeptide, mature toxin) found in the venom gland. Thus, the development of a specialized venom duct, where different toxin types are regionally produced, was a key functional innovation to allow separate venoms to be injected for predation and defence. At this stage, it is unclear if venom duct specialization arose from migration of specialized secretory cells from one section of the venom duct to another, or whether varying transcriptomic regulation explains the distinct venom peptide expression profiles in different duct regions. While proximal–distal heterogeneity in toxin production along the venom duct of Conus textile has been reported previously [16] , [17] , its role was not identified. Our results now reveal that stimulus-dependent spatiotemporal release of toxins from different segments of the venom duct can generate functionally and biochemically distinct predation- and defence-evoked venoms that are presumably under separate neuronal control (see Fig. 3f ). Stimulus-dependent release of venom likely explains the occasional ‘dry stings’, which correspond to injection of venom devoid of peptidic toxins [18] . Regional specialization of toxin production also explains early observations that injection of extracts of distal duct venom had no effect on mice while extracts of proximal duct venom were lethal [19] , and is supported by recent transcriptomic analysis that found distinct messenger RNA expression patterns in distal and proximal C. geographus venom duct [20] . While venom diversification in cone snails has only been associated with dietary specialization [21] , our study reveals that both predatory and defensive strategies contribute to venom evolution by rapidly accumulating variations under the influence of positive Darwinian selection, often in an episodic manner. From recent studies on the evolutionary relationships of Conus species, it is now generally accepted that vermivory was the ancestral feeding mode from which specialized diets (that is, molluscivory and piscivory) arose. Evidence includes phylogenetic analyses of conotoxins expressed by piscivorous species that were likely derived from a set of loci that was present in the ancestral vermivorous lineages [22] , and the observation that some piscivorous species consume worms as juveniles [23] . However, no satisfactory hypothesis has been proposed to explain the shift from worm to mollusk or fish prey. Our results now suggest an unexpected evolutionary path to diet diversification in Conidae. We propose that defence-evoked venom originally evolved in worm-hunting species to protect against predation by fish and cephalopods was repurposed in the predatory venom to facilitate the evolution of piscivorous and molluscivorous feeding strategies ( Fig. 4c ). In support, a predation-evoked sting from the non-piscivorous species C. textile injected into fish was not paralytic ( Supplementary Movie 4 ), whereas a defensive sting produced rapid paralysis ( Supplementary Movie 5 ). Similarly, the fish-hunting C. obscurus rapidly paralyses fish, but using a ‘hook-and-line’ predatory strategy, which may have evolved from ancestral defence-evoked venoms ( Supplementary Movie 6 ). Escape from predation is essential for animal survival. Among the diverse range of evolved adaptations [24] , the specific defensive envenomation strategy employed by cone snails appears among the most remarkable. It is well known that some venomous animals can ‘metre’ their venom use based on the size of the prey or the intensity of the threat [25] , [26] . For example, scorpions use a toxin-poor ‘prevenom’ primarily to subdue small prey or deter low-level threats and only use their toxin-rich ‘true venom’ for high-level threats [27] . Such behavioural adaptations likely evolved to limit venom expenditure, as the production of venom toxins is metabolically expensive [28] . Our results demonstrate that venomous animals can modify the toxin composition of venom according to a predatory or defensive stimulus, in an interchangeable manner. In conclusion, the separate defensive envenomation strategy employed by cone snails is a remarkable adaptation, changing our understanding of the biology, evolution and toxin diversification mechanisms in Conidae. This knowledge will also rationalize approaches to discover novel vertebrate-active conotoxins found preferentially in defence-evoked venom and proximal venom duct peptides, and prey-specific conotoxins found preferentially in predation-evoked venoms and distal venom duct peptides. Moreover, since the defensive use of venom is a general feature of most venomous animals, its evolutionary impact on venom diversification remains to be assessed in phylogenetically unrelated groups. Indeed, snakes and spiders can control venom expenditure and produce pain-inducing toxins to deter predators [29] , [30] . Recently, regionalization of toxin production has been shown in sea anemone [31] , indicating that deployment of separate venoms might not be restricted to cone snails. Based on these observations, the evolution of specialized defensive venoms is predicted to be more important and widespread in other venomous animals than previously recognized, especially those with diversified diets. We propose that this specialization has allowed cone snails to repurpose conotoxins found in defensive venom to protect against fish and cephalopod threats to allow these predatory groups to become prey for piscivorous and molluscivous cone snails. Venom collection All cone snails used in this study have been collected from Queensland coastal waters under a research permit issued from the Great Barrier Reef Marine Park (G10/33243.1). Cone snails were held in aquaria (5 weeks to 2 years) at a temperature maintained between 24–28 °C and a 12:12 light–dark cycle. Following each milking, the collecting tube was briefly centrifuged, lyophilized and stored at –20 °C until use. Predation-evoked venom samples from the fish-hunting cone snails C. geographus and C. obscurus were obtained as previously described [32] . Briefly, a live fish is used to lure the cone snail and elicit a predatory behaviour with extension of the proboscis. A microcentrifuge tube covered with parafilm and a piece of fish tail is then presented at the tip of the proboscis, and upon contact with fish tissue, predation-evoked venom is forcefully injected through the hollow harpoon-like radula into the collecting tube. To obtain defensively injected venom samples, a novel milking procedure was developed to engage the animal in a defensive mode. The procedure involved removing the cone snail from the tank and applying light pressure to the shell with long forceps until it was provoked to extend its proboscis. Once the proboscis was extended, a collecting tube covered with parafilm was presented to the tip of the proboscis until stinging occurred. Depending on the cone snail, several attempts were often required to trigger a stinging response and the delivery of venom into the tube. Owing to the serious health hazard associated with C. geographus envenomation, this milking procedure should only be attempted by persons fully aware of and protected from the risk of an accidental sting (for example, wearing thick gloves and carefully manipulating the snails with long forceps). The predation-evoked venom from mollusk-hunting cone snails C. marmoreus and C. victoriae were collected as previously described [14] . Like other mollusk hunters, C. marmoreus and C. victoriae usually inject their prey multiple times with venom during a single feeding event. Therefore, these species could be challenged in alternating predatory and defensive modes during a single milking session. The defence-evoked venom was obtained as outlined for C. geographus , except that repeated light pinching the foot of the animal was required to induce a similar defensive behaviour. For the worm-hunting cone snails C. planorbis and C. coronatus, we used the predator C. marmoreus to trigger a defensive behaviour and initiate extension of the proboscis. The defence-evoked venom was then collected as described for C. geographus . RNA extraction and transcriptome sequencing The transcriptome of a pool of C. geographus venom ducts was recently published [20] . This study provides additional support to earlier proteomic and toxicity studies that suggested the presence of distinct venom-expression patterns along the duct, with disorientating and paralytic venoms expressed in different regions. To evaluate the possible contribution of different organs to conotoxin production, a single adult specimen of C. geographus collected from the Great Barrier Reef (Queensland, Australia) and measuring 10 cm was dissected on ice to remove the venom duct, salivary gland and radular sac. Samples were placed separately into 1 ml of TRIZOL reagent (Invitrogen) and total RNA extracted following the manufacturer’s instructions to yield ~400 ng of purified messenger RNA from each tissue (Dynabeads mRNA DIRECT kit, Invitrogen). A cDNA library was constructed by fragmenting the RNA, synthesis of double-stranded cDNA, fragment end repair, preparation of AMPure beads, ligation of adaptors and removal of small fragments, followed by quantitation and quality assessment. cDNA sequencing was carried out on a Roche 454 GS FLX Titanium sequencer. The three tissue samples were run together on a full plate, using a unique barcode for each sample. Transcriptomic analysis Sorting of raw cDNA reads obtained from transcriptome sequencing was performed with ConoSorter, a standalone programme developed in house to classify conopeptides into gene superfamilies and classes [33] . After translating the nucleic acid sequences in the six reading frames using the universal genetic code, the algorithm isolates the corresponding CDS regions before matching the sequences against complementary regular expressions and profile Hidden Markov Models built from separate signal, pro- and mature conopeptide regions. The programme then searches the ConoServer database [34] for known precursor sequences and generates additional information relative to the hits obtained (frequency of sequences in the raw data set, percentage of hydrophobicity of the amino-terminal region, sequence length, number of cysteines, scores and bias) in order to sort the reads. C. geographus transcriptomic sequences with at least duplicate reads ( n =2) and >50 amino acids were sorted into superfamilies and their corresponding template cDNA sequence retrieved for the subsequent molecular evolution analysis. Proteomic analyses Five adult specimens of C. geographus collected from the Great Barrier Reef (Queensland, Australia) were held in an aquarium for several weeks for predation- and defence-evoked venom collection. Two specimens were killed for tissue-based proteomic studies. Dissection was carried out on ice and the venom duct removed and divided into 12 equal 1.2-cm sections. The content of each fraction was squeezed from the duct and diluted with 0.1% formic acid. The salivary glands and radular sac were extracted with 0.1% formic acid and stored at –20 °C prior to use. Liquid chromatography and electrospray mass spectrometry was performed on the AB Sciex 5600 TF and AB Sciex QSTAR Pulsar as previously described [14] , [35] . Briefly, the predation- and defence-evoked venom samples, the 12 sections of the dissected venom, as well as the extracts from the salivary gland and the radular sac were directly subjected to LC-ESI-MS in order to obtain a complete mass list of underivatized peptides. Information-dependent acquisition was performed on the reduced, reduced/alkylated and enzymatically digested venom samples. A sequence database comprising the entire raw cDNA reads from this transcriptomic project was used to match MS/MS data with transcriptomic sequences utilizing Protein Pilot 4 software. The detected peptide fragments (confidence value >99) were manually inspected and validated. The extracts of the 12 duct sections were analysed using an Ultraflex III TOF-TOF (time-of-flight) mass spectrometer (Bruker Daltonics, Bremen, Germany) equipped with a 200 Hz all-solid-state laser (SmartBeam) and controlled by the FlexControl 2.4 software package. Our analytes have molecular weights between 1,000 kDa and 10,000 kDa and therefore the Ultraflex III was operated in both linear-positive and reflectron-positive mode using CHCA as a matrix. Spectra calibration was performed externally using a peptide calibration mixture (206195, Bruker Daltonics, Bremen, Germany). A CHCA solution was made by the dilution of acetone saturated with CHCA 1 in 10 with an acetone:acetonitrile:water (6:3:1) solution. The raw samples were diluted 1 in 100 with 0.1% TFA, and 2 μl of diluted matrix solution mixed with 1 μl sample and spotted onto a polished steel target. For all samples, 400 shots were acquired using a random walk function at a laser frequency of 200 Hz and saved, with 10 replicates of each sample averaged. Data were loaded into Clinprot Tools (Bruker Daltonics, Bremen, Germany) to visualize the 12 individual duct sections in ‘gel view’ using a colorimetric gradient to show the abundance of the components in respective fractions. Histology Cone snails were fixed with paraformaldehyde, dehydrated using ethanol and processed using a Sakura Tissue-Tek VIP processor with a programme of 30 min xylene clear, and 4 × 30 min paraffin penetrations. The processed animals were then prepared into paraffin blocks (Shandon Histocentre 3) and cut at ~5 μm using a Leica RM2235 microtome. Glass slides (Lomb Menzel Glaser) were used during histological sectioning. Sections of paraformaldehyde-fixed animals were cut at ~5 μm, floated out on a water bath, incubated in a Thermoline hot air drier at 60 °C for 30 min and stained according to the following protocol. Sections were de-paraffinized with xylene, rehydrated from ethanol back to water and then stained using Weigert haematoxylin for 10 min. Following this, the slides were washed in running water, differentiated in acid alcohol and Scott’s tap water. The slides were then washed in running water, rinsed in distilled water and stained with Gomori’s trichrome for 20 min. Finally, the slides were rinsed with 0.5% acetic acid, distilled water and dehydrated with alcohol through to xylene, before being cover-slipped. The muscle fibres stain red, collagen stains green and the nuclei stain blue/black. Bioassay at human Ca v , Na v and nAChR in SH-SY5Y cells Predation- and defence-evoked venoms (1 mg each) were separated on a C 18 analytical column (Grace Vydac) eluted at 1 ml min −1 with an UltiMate 3000 LC system (Dionex) and 1-min fractions collected using and a FC 204 fraction collector (Gilson). The activity of each fraction was assessed using high-throughput Ca 2+ imaging assays, as previously described [36] . In brief, SH-SY5Y cells (European Collection of Cell Cultures) were maintained in RPMI medium (Invitrogen, Australia) supplemented with 15% fetal bovine serum and L -glutamine and passaged every 3–5 days using 0.25% trypsin/EDTA (Invitrogen). SH-SY5Y cells were plated at a density of 35,000–50,000 cells per well on 384-well black-walled imaging plates and cultured for 48 h. Fluorescent responses (excitation 470–495 nm; emission 515–575 nm) were assessed using the FLIPR Tetra fluorescent plate reader (Molecular Devices) after 30-min incubation with fluorescent Ca 2+ dye (Calcium 4 No Wash dye, Molecular Devices) diluted in physiological salt solution (composition in mM: NaCl 140, glucose 11.5, KCl 5.9, MgCl 2 1.4, NaH 2 PO 4 1.2, NaHCO 3 5, CaCl 2 1.8, HEPES 10). The equivalent of 50 μg crude venom was added 5 min prior to stimulation of endogenously expressed Na v , Ca v and nAChR isoforms. To assess activity at Na v isoforms endogenously expressed in SH-SY5Y cells (Na v 1.2 and Na v 1.7), SH-SY5Y cells were stimulated with veratridine (50 μM), while activity at Ca v 2.2 channels was assessed in the presence of nifedipine (10 μM) after stimulation with KCl (90 mM) and CaCl 2 (5 mM). Nicotine (30 μM) was used to activate endogenously expressed human α3β2 and α3β4 nAChR, while endogenously expressed human α7 nAChR were activated using the α7 nAChR agonist choline (30 μM) in the presence of the allosteric modulator PNU120596 (10 μM, Sigma-Aldrich). Responses were normalized to baseline using ScreenWorks 3.2.0.14 (Molecular Devices) and the maximum increase in fluorescence for each predation-evoked venom fraction was plotted relative to the corresponding defence-evoked venom fraction using GraphPad Prism 5.03, in order to identify fractions with differential activity between both modes. Fish bioassay Wild-type zebrafish ( Danio rerio ) reared in the laboratory for 6–10 months were injected intramuscularly with 5 μl of saline solution (control) or serial dilutions of C. geographus predation- or defence-evoked venoms using a Hamilton syringe. Fish were then observed for signs of paralysis over 10 min in a 5 l swim tunnel (Loligo Systems ApS, Denmark) operated at 250 revolutions per minute. The onset of paralysis was recorded as the time fish drifted to the opposite end of the tunnel, with unaffected and saline-injected fish able to swim into the current without signs of exhaustion for more than 1 h. Time of paralysis versus quantity of venom injected (predatory or defensive) was used to calculate the effective dose (ED 50 ) in GraphPad Prism 5.03. Ethical approval for zebrafish experiments was obtained from the University of Queensland animal ethics committee (IMB/066/12/ARC/NHMRC). Molecular evolution analyses To overcome the effects of recombination on the phylogenetic and evolutionary interpretations, we employed Single Breakpoint algorithms implemented in the HyPhy package and assessed recombination on all the toxin forms examined in this study [37] . When potential breakpoints were detected using the small sample Akaike information Criterion (AICc), the sequences were compartmentalized before conducting selection analyses. The influence of natural selection on various C. geographus and C. marmoreus toxin types was evaluated using maximum-likelihood models implemented in CODEML of the PAML package [38] . We employed site-specific models that estimate positive selection statistically as a non-synonymous to synonymous nucleotide substitution rate ratio (ω) significantly greater than 1. We compared likelihood values for three pairs of models with different assumed ω distributions as no a priori expectation exists for the same: M0 (constant ω rates across all sites) versus M3 (allows ω to vary across sites within ‘n’ discrete categories, n ≥3); M1a (a model of neutral evolution) where all sites are assumed to be either under negative (ω<1) or neutral selection (ω=1) versus M2a (a model of positive selection), which, in addition to the site classes mentioned for M1a, assumes a third category of sites; sites with ω>1 (positive selection) and M7 (Beta) versus M8 (Beta and ω) and models that mirror the evolutionary constraints of M1 and M2 but assume that ω values are drawn from a beta distribution. Only if the alternative models (M3, M2a and M8: allow sites with ω>1) show a better fit in Likelihood Ratio Test relative to their null models (M0, M1a and M7: do not allow sites to have ω>1), are their results considered significant. Likelihood Ratio Test is estimated as twice the difference in maximum-likelihood values between nested models and compared with the χ 2 distribution with the appropriate degree of freedom (the difference in the number of parameters between the two models). The Bayes empirical Bayes (BEB) approach was used to identify amino acids under positive selection by calculating the posterior probabilities that a particular amino acid belongs to a given selection class (neutral, conserved or highly variable). Sites with greater posterior probability (PP≥95%) of belonging to the ‘ω>1 class’ were inferred to be positively selected. Fast, Unconstrained Bayesian AppRoximation [39] implemented in HyPhy [40] was employed to detect sites evolving under the influence of pervasive diversifying and purifying selection. Mixed Effects Model Evolution (MEME) [41] was also used to detect episodic burst of selection. To reveal the proportion of sites under different regimes of selection, an evolutionary fingerprint analysis was carried out using the evolutionary selection distance algorithm implemented in datamonkey [42] . We further utilized branch-site Random Effects Likelihood [43] to identify lineages affected by episodic selection. Accession codes : cDNA sequences have been deposited in the DDBJ database under accession codes AB910766 to AB910895 . How to cite this article : Dutertre, S. et al. Evolution of separate predation- and defence-evoked venoms in carnivorous cone snails. Nat. Commun. 5:3521 doi: 10.1038/ncomms4521 (2014).